Topological superfluids with finite-momentum pairing and Majorana fermions Majorana fermions (MFs), quantum particles that are their own antiparticles, are not only of fundamental importance in elementary particle physics and dark matter, but also building blocks for fault-tolerant quantum computation. Recently MFs have been intensively studied in solid state and cold atomic systems. These studies are generally based on superconducting pairing with zero total momentum. On the other hand, finite total momentum Cooper pairings, known as Fulde–Ferrell (FF) Larkin–Ovchinnikov (LO) states, were widely studied in many branches of physics. However, whether FF and LO superconductors can support MFs has not been explored. Here we show that MFs can exist in certain types of gapped FF states, yielding a new quantum matter: topological FF superfluids/superconductors. We demonstrate the existence of such topological FF superfluids and the associated MFs using spin–orbit-coupled degenerate Fermi gases and derive their parameter regions. The implementation of topological FF superconductors in semiconductor/superconductor heterostructures is also discussed. Topological superconductors and superfluids are exotic quantum matters that host topological protected excitations, such as robust edge modes and Majorana fermions (MFs) with non-Abelian exchange statistics [1] . MFs are important not only because of their fundamental role in elementary particle physics and dark matters [2] , but also because of their potential applications in fault-tolerant topological quantum computation [3] . Recently some exotic systems, such as ν =5/2 fractional quantum Hall states [3] , chiral p -wave superconductors/superfluids [3] , heterostructure composed of s -wave superconductors and semiconductor nanowires (nanofilms) or topological insulators [4] , [5] , [6] , [7] , [8] , [9] , [10] and so on, have been proposed as systems supporting MFs. Following the theoretical proposals, exciting experimental progress for the observation of MFs has been made recently in semiconductor [11] , [12] , [13] , [14] or topological insulator heterostructures [15] , although unambiguous experimental evidence for MFs is still lacked. These theoretical and experimental studies are based on the superconducting Cooper pairing ( s -wave or chiral p -wave) with zero total momentum, that is, the pairing is between two fermions with opposite momenta k and − k (denoted as Bardeen-Cooper-Schrieffer (BCS) pairing hereafter). On the other hand, the superconducting pairing can also occur between fermions with finite total momenta (pairing between k and − k + Q ) in the presence of a Zeeman field, leading to spatially modulated superconducting order parameters in real space, known as Fulde–Ferrell (FF) and Larkin–Ovchinnikov (LO) states. The FF and LO states were first predicted in 1960s [16] , [17] , and now are a central concept for understanding exotic phenomena in many different systems [18] , [19] , [20] , [21] , [22] , [23] . A natural question to ask is whether MFs can also exist in an FF or LO superconductor or superfluid? In this article, we propose that FF superconductors/superfluids may support MFs if they possess two crucial elements: gapped bulk quasi-particle excitations and non-trivial Fermi surface topology. These new quantum states are topological FF superconductors/superfluids. In this context, traditional gapless FF states induced by a large Zeeman field do not fall into this category. Here we propose a possible platform for the realization of topological FF superfluids using two-dimensional (2D) or one-dimensional (1D) spin–orbit (SO)-coupled degenerate Fermi gases subject to in-plane and out-of-plane Zeeman fields. Recently, the SO coupling and Zeeman fields for cold atoms have already been realized in experiments [24] , [25] , [26] , [27] , [28] , which provide a completely new avenue for studying topological superfluid physics. It is known that SO-coupled degenerate Fermi gases with an out-of-plane Zeeman field support MFs with zero total momentum pairing [29] , [30] , [31] , [32] . We find in suitable parameter regions the in-plane Zeeman field can induce the finite total momentum pairing [33] , [34] , [35] , [36] , [37] , while still keeps the superfluid gapped and preserves its Fermi surface topology. The region for topological FF superfluids depends not only on the chemical potential, pairing strength, but also on the SO coupling strength, total momentum and effective mass of the Cooper pair, as well as the orientation and magnitude of the Zeeman field, thus greatly increases the tunability in experiments. Finally, the potential implementation of the proposal in semiconductor/superconductor heterostructures is also discussed. System and Hamiltonian Consider an SO-coupled Fermi gas in the xy plane with the effective Hamiltonian where , k =( k x , k y ), α is the Rashba SO coupling strength, h =( h x , 0, h z ) is the Zeeman field and is the Pauli matrices. describes the s -wave scattering interaction, where is the scattering interaction strength, E b is the binding energy and k 1 + k 2 = k 3 + k 4 due to the momentum conservation. In experiments, 2D degenerate Fermi gases can be realized using a 1D deep optical lattice along the third dimension [38] , [39] , where the tunnelling between different layers is suppressed. The pseudospins of atoms are defined through atomic hyperfine ground states. By transferring Raman photons between two hyperfine ground states, an effective 1D SO coupling (used below) has been created in experiments for both bosonic and fermionic atoms [24] , [25] , [26] , [27] , [28] , where the effective in-plane and out-of-plane Zeeman fields can be tuned independently by varying the detuning and intensity of the Raman coupling lasers. The schemes for the realization of 2D Rashba SO coupling are similar, but involve more laser beams, as proposed in several different theoretical schemes [40] , [41] , [42] . Without in-plane Zeeman field h x , the Fermi surface is symmetric around k =0, and the superfluid pairing is between atoms with opposite momenta k and − k ( Fig. 1b ). Although with both h x and SO coupling, the Fermi surface becomes asymmetric along the y direction (see Fig. 1a,c ), and the pairing can occur between atoms with momenta k and − k + Q . In real space, such a finite total momentum pairing may lead to a FF-type order parameter Δ( x )=Δ e i Q · x with a single FF momentum Q =(0, Q y ) that is parallel to the deformation direction of the Fermi surface, as found in recent real [37] and momentum [33] , [34] , [35] space calculations. Note that k and − k + Q for the FF-type Cooper pairs may not stay simultaneously on the Fermi surface for all k . However, the pairing between them is still effective because the pairing can occur not only exactly on the Fermi surface, but also near the Fermi surface with an energy width determined by the order parameter Δ, which, for cold atomic systems, can be comparable to the Fermi energy [43] . The basic picture presented in Fig. 1 still holds in this case. The energies of the superfluids with total momentum Q and − Q are non-degenerate; therefore, FF phase with a single Q , instead of LO phase (Δ( x )=Δcos( Q·x )) where pairing occurs at both ± Q , is more energetically favourable for the parameters considered here. 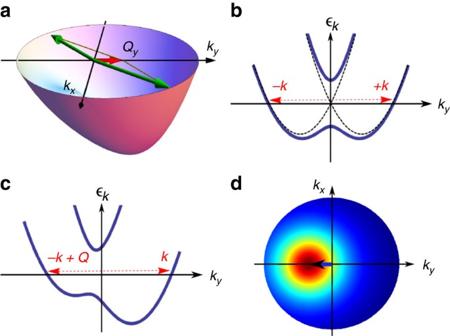Figure 1: Single-particle band structure and Berry curvature. (a) Energy dispersion of the lower band and an illustration of the FF-type of Cooper pairing. The green arrows represent the momenta of a Cooper pair of two atoms on the asymmetric Fermi surface. The red arrow represents the total finite momentum of the paring, which is along the deformation direction of the Fermi surface. Note thatkand −k+Qmay not be along the same line in 2D. (b) Symmetric band structure withhx=0, which supports zero total momentum pairing. Dashed lines represent the band dispersion withhz=0. (c) Asymmetric band structure withhx≠ 0, which supports FF state with finite-momentum pairing. Onlykx=0 plane is shown in (b) and (c). (d) Berry curvature of the lower band, whose peak is shifted from the origin byhx/αalong thekydirection. Figure 1: Single-particle band structure and Berry curvature. ( a ) Energy dispersion of the lower band and an illustration of the FF-type of Cooper pairing. The green arrows represent the momenta of a Cooper pair of two atoms on the asymmetric Fermi surface. The red arrow represents the total finite momentum of the paring, which is along the deformation direction of the Fermi surface. Note that k and − k+Q may not be along the same line in 2D. ( b ) Symmetric band structure with h x =0, which supports zero total momentum pairing. Dashed lines represent the band dispersion with h z =0. ( c ) Asymmetric band structure with h x ≠ 0, which supports FF state with finite-momentum pairing. Only k x =0 plane is shown in ( b ) and ( c ). ( d ) Berry curvature of the lower band, whose peak is shifted from the origin by h x / α along the k y direction. Full size image The dynamics of the system can be described by the following Bogliubov-de Gennes (BdG) Hamiltonian in the mean-field level, where the Nambu basis is chosen as . The gap, number and momentum equations are solved self-consistently to obtain Δ, μ and Q (see Methods), through which we determine different phases. Physical mechanism for topological FF phase Without SO coupling, the orientation of the Zeeman field does not induce any different physics due to SO(2) symmetry. The presence of both h x and SO coupling breaks this SO(2) symmetry, leading to a Fermi surface without inversion symmetry, see Fig. 1a–c . Here, h x deforms the Fermi surface, leading to FF Cooper pairings, whereas h z opens a gap between the two SO bands, making it possible for the chemical potential to cut a single Fermi surface for the topological FF phase. The Berry curvature of the lower band reads as Note that h x shifts the peak of Berry curvature from k =0 to (0, − h x / α ) (denoted by an arrow in Fig. 1d ). When atoms scatter from k to k ′ on the Fermi surface, they pick up a Berry phase, whose accumulation around the Fermi surface θ = ∬ d 2 k Ω k ≈ π . Such Berry phase modifies the effective interaction from s -wave ( is a constant) to s -wave plus asymmetric p -wave on the Fermi surface. Here we recover the well-known chiral p x + ip y pairing [29] in the limit h x =0. The in-plane Zeeman field here creates an effective s -wave pairing component (although still hosts MFs), and the effective pairing is reminiscent to the ( s + p )-wave pairing in some solid materials [44] . Parameter region for MFs The BdG Hamiltonian (2) satisfies the particle-hole symmetry , where Λ= iσ y τ y , is the complex conjugate operator and Ξ 2 =1. The parameter region for the MFs is determined by the topological index , where Pf is the Pfaffian of the skew matrix Γ= H BdG ( 0 )Λ. corresponds to the topologically non-trivial (trivial) phase [45] . The topological phase exists when where and . E g =min( E k , s ) defines the bulk quasi-particle excitation gap of the system with E k , s as the particle branches of the BdG Hamiltonian (2). The first condition reduces to the well-known in BCS topological superfluids [6] , [7] , [11] , [12] , [13] , [14] , [31] . The last condition ensures the bulk quasi-particle excitations are gapped to protect the zero-energy MFs in the topological regime. The SO coupling and the FF vector shift the effective in-plane Zeeman field and the chemical potential. In contrast, in the BCS topological superfluids, the SO coupling strength, although required, does not determine the topological boundaries. Our system therefore provides more knobs for tuning the topological phase transition. To further verify the topological condition in equation (5), we calculate the Chern number in the hole branches in the gapped superfluids [45] , and confirm =+1 when equation (5) is satisfied and =0 otherwise. Here is the Chern number, is the Berry curvature [46] , and is the eigenstate of two hole bands of the BdG Hamiltonian (2). The transition from non-topological to topological phases defined by equation (5) can be better understood by observing the close and reopen of the excitation gap E g , which is necessary to change the topology of Fermi surface. In Fig. 2 , we plot the change of E g along with the order parameter |Δ|, the chemical potential μ and the FF vector Q as a function of Zeeman fields. For a fixed h x but increasing h z , E g may first close and then reopen ( Fig. 2a ), signalling the transition from non-topological to topological gapped FF superfluids ( Q y is finite for all h z , see Fig. 2b ). For a fixed h z , the superfluid is gapped and Q y h x for a small h x (see Fig. 2d ), thus any small h x can transfer the gapped BCS superfluids at h x =0 to FF superfluids. However, such a small h x does not destroy the bulk gap of BCS superfluids (topological or non-topological), making gapped topological FF superfluids possible when the system is initially in topological BCS superfluids without h x . With increasing h x ( Fig. 2c ), E g may first close but does not reopen immediately, signalling the transition from gapped FF superfluids to gapless FF superfluids. For a small h z =0.2 E F , further increasing h x to , E g reopens again ( Fig. 2c ), signalling the transition from gapless FF to gapped topological FF superfluids. In this regime, , which is not small. For a strong enough Zeeman field, the pairing may be destroyed and the system becomes a normal gas. 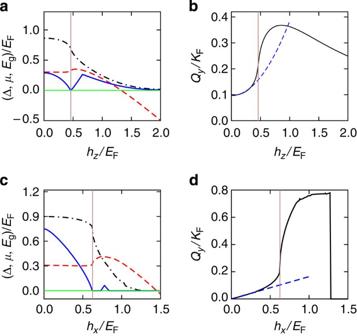Figure 2: Effects of Zeeman fields. The order parameter Δ (dash-dotted black line), chemical potentialμ(dashed red line), bulk quasi-particle gapEg(solid blue line), and FF vectorQy(solid black line) are plotted as a function of out-of-plane Zeeman fieldhz(a,b) and in-plane Zeeman fieldhx(c,d), respectively. The energy unit for Δ,μ, andEgisEF. The dashed blue lines in (b) and (d) are the best fitting with quadratic and linear functions in the small Zeeman field regime, respectively. In (a) and (b),hx=0.2EF, whereas in (c) and (d),hz=0.2EF. Other parameters areEb=0.4EF,αKF=1.0EF. The vertical lines mark the points where the Pfaffian changes the sign. Figure 2: Effects of Zeeman fields. The order parameter Δ (dash-dotted black line), chemical potential μ (dashed red line), bulk quasi-particle gap E g (solid blue line), and FF vector Q y (solid black line) are plotted as a function of out-of-plane Zeeman field h z ( a , b ) and in-plane Zeeman field h x ( c , d ), respectively. The energy unit for Δ, μ , and E g is E F . The dashed blue lines in ( b ) and ( d ) are the best fitting with quadratic and linear functions in the small Zeeman field regime, respectively. In ( a ) and ( b ), h x =0.2 E F , whereas in ( c ) and ( d ), h z =0.2 E F . Other parameters are E b =0.4 E F , αK F =1.0 E F . The vertical lines mark the points where the Pfaffian changes the sign. Full size image The complete phase diagrams are presented in Fig. 3 . As Q y and h x have the same sign, the phase diagrams show perfect symmetry in the h x − h z plane. The BCS superfluids can only be observed at h x =0, hence are not depicted. With increasing SO coupling strength, the topological FF phase is greatly enlarged through the expansion to the normal gas phase. For a small SO coupling ( Fig. 3a ), a finite h z is always required to create the topological FF phase; In the intermediate regime ( Fig. 3b ), we find an interesting parameter regime where the topological FF phase can be reached with an extremely small h z around . However, the topological FF phase can never be observed at h z =0, as analysed before from the Berry curvature and Chern number. From Fig. 3a,b , we see that the topological gapped FF phase can be mathematically regarded as an adiabatic deformation of the topological BCS superfluids by an in-plane Zeeman field, although their physical meaning are totally different. In Fig. 3c,d , we see that the gapless FF phase can be observed at small binding energy and small h z , whereas for large enough binding energy, the system can be either topological or non-topological gapped phases. In this regime, , where , and , thus h z E b is required to close and reopen E g (see Fig. 3c,d ). 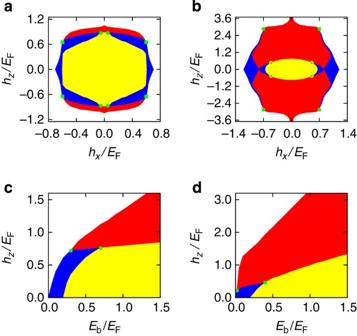Figure 3: Phase diagram of the FF superfluid. The phases are labelled with different colours: topological gapped FF superfluid (red), non-topological gapped FF superfluid (yellow), gapless FF superfluid (blue) and normal gas (white). Other parameters are: (a)Eb=0.4EF,αkF=0.5EF; (b)Eb=0.4EF,αkF=1.0EF; (c)hx=0.5EF,αkF=0.5EF; and (d)hx=0.5EF,αkF=1.0EF. The symbols in each panel are the tricritical points. Figure 3: Phase diagram of the FF superfluid. The phases are labelled with different colours: topological gapped FF superfluid (red), non-topological gapped FF superfluid (yellow), gapless FF superfluid (blue) and normal gas (white). Other parameters are: ( a ) E b =0.4 E F , αk F =0.5 E F ; ( b ) E b =0.4 E F , αk F =1.0 E F ; ( c ) h x =0.5 E F , αk F =0.5 E F ; and ( d ) h x =0.5 E F , αk F =1.0 E F . The symbols in each panel are the tricritical points. Full size image The tricritical points marked by symbols in Fig. 3 are essential for understanding the basic structure of the phase diagram. Along the h z axis, the system only supports gapped BCS superfluids (topological or non-topological) and normal gas [31] , whereas along the h x axis the system only supports trivial FF superfluids and normal gas [33] , [34] , [35] . So the adiabatic connection between the topological BCS superfluids and trivial FF phases is impossible, and there should be some points to separate different phases, which are exactly the tricritical points. In our model, the transition between different phases is the first-order process. The existence of tricritical point here should be in stark contrast to the tricritical point at finite temperature in the same system without SO coupling, which arises from the accidental intersection of first- and second-order transition lines [23] . Therefore, the tricritical points in Fig. 3 cannot be removed, although their specific positions vary with the system parameters. Chiral edge modes The topological FF superfluids support exotic chiral edge modes. To see the basic features more clear, we consider the same model in a square lattice with the following tight-binding Hamiltonian: where , and with . Here, c iσ denotes the annihilation operator of a fermionic atom with spin σ at site i =( i x , i y ). Hereafter, we use t =1 as the basic energy unit. For more details, see Methods. In the following, we only present the chiral edge states in the topological gapped FF superfluid regime, and assume Δ i = Δ. We consider a 2D strip with width W =200, and the results for the strip along x and y directions in the topological FF phase are presented in Fig. 4 . Similarly, here the energy spectrum is obtained after a gauge transformation to remove the order parameter spatial dependence (see Methods). 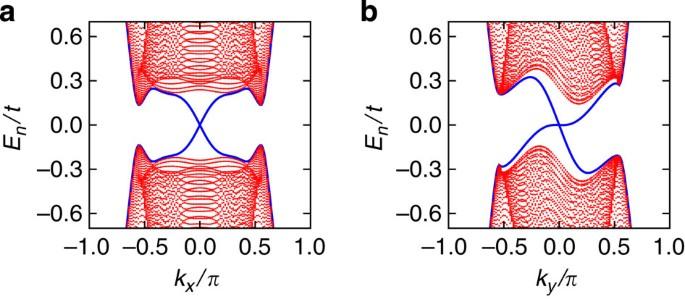Figure 4: Chiral edge states of topological FF phases in a 2D strip. The strip is along thexdirection in (a) andydirection in (b). The parameters areμ= − 4t,α=2.0t, Δ=0.3t,hz=1.2t,hx=0.5tandQy=0.4. The linear dispersion of the edge states reads as Figure 4: Chiral edge states of topological FF phases in a 2D strip. The strip is along the x direction in ( a ) and y direction in ( b ). The parameters are μ = − 4 t , α =2.0 t , Δ=0.3 t , h z =1.2 t , h x =0.5 t and Q y =0.4. Full size image where L and R define the left and right edges of the strip, and v L and v R are the corresponding velocities. We have also confirmed that the wavefunctions of the edge states are well localized at two edges. For a strip along the x direction, the particle-hole symmetry as well as the inversion symmetry ( k x →− k x ) ensure that the eigenenergies of equation (6) always come in pairs ( E k ,− E k ), thus v R = v L ( Fig. 4a ). However, when the strip is along the y direction (parallel to the FF momentum Q and the in-plane Zeeman field h x ), the eigenenergies no longer come in pairs, therefore v R ≠ v L ( Fig. 4b ). Note that the asymmetric spectrum along the k y direction originates from the intrinsic inversion symmetry breaking ( k y →− k y ) of the system, and cannot be restored by simply changing the observation frame. There are two factors that contribute to the asymmetric spectrum: (i) the SO coupling and in-plane Zeeman field, which distort the single-particle band as shown in Fig. 1c ; (ii) the FF momentum Q , which shifts particle and hole bands along different directions. Both of them lead to asymmetric edge velocities. A careful examination shows that the overall edge spectrum is still asymmetric with both factors taken into account because of the intrinsic inversion symmetry breaking. The velocity difference v R − v L depends on many different parameters ( α , h x , Q and so on), and there is no simple relation between v R − v L and Q . In fact, v R − v L is still non-zero even when Q is forced to be zero. The Chern number =1 in our lattice model, thus only one pair of chiral edge states can be observed. MFs in 1D chain Topological FF superfluid and associated MFs can also be observed in 1D SO-coupled Fermi gas when the Hamiltonian (6) is restricted to 1D chain. In this case, the system is characterized by a Z 2 invariant, which can be determined using the similar procedure as discussed above. The only difference is that now not only k =0, but also k = π need be taken into account (see Methods). In Fig. 5a , we see Majorana zero-energy state protected by a large gap ( ) emerges in a suitable parameter region. The superfluid order parameter ( Fig. 5b ) has the FF form in the bulk and responses to the boundary in the length scale of the healing length v F /Δ, which is estimated to be lattice sites for the parameters used in Fig. 5b , agreeing with the numerical results. The local Bogoliubov quasi-particle operator , where the zero-energy wavefunction satisfies at the left edge and at the right edge (see Fig. 5c ). This state supports two local MFs at two edges, respectively [6] . 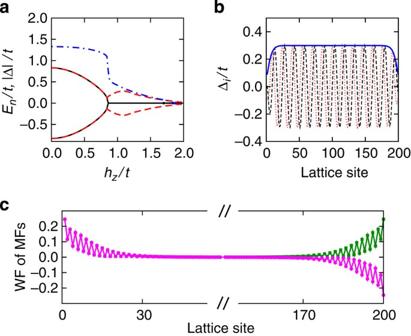Figure 5: Majorana fermions in a 1D chain. (a) Plot of the BdG quasi-particle excitation energies ±E2(dashed red line), ±E1(solid black line), and the order parameter (dash-dotted blue line). (b) The spatial profile of the FF-type order parameter obtained self-consistently. The dotted red and dashed black lines correspond to the real and imaginary parts of Δi. The solid blue line represents |Δi|. (c) The wavefunction (WF) of the Majorana zero-energy state (U↑,V↑) in the 1D chain. Green line,U↑; red line,V↑. (U↓,V↓) is similar but with different amplitudes. The parameters areα=2.0t,hx=0.5t,hz=1.2t,U=4.5tandμ=−2.25t. Figure 5: Majorana fermions in a 1D chain. ( a ) Plot of the BdG quasi-particle excitation energies ± E 2 (dashed red line), ± E 1 (solid black line), and the order parameter (dash-dotted blue line). ( b ) The spatial profile of the FF-type order parameter obtained self-consistently. The dotted red and dashed black lines correspond to the real and imaginary parts of Δ i . The solid blue line represents |Δ i |. ( c ) The wavefunction (WF) of the Majorana zero-energy state ( U ↑ , V ↑ ) in the 1D chain. Green line, U ↑ ; red line, V ↑ . ( U ↓ , V ↓ ) is similar but with different amplitudes. The parameters are α =2.0 t , h x =0.5 t , h z =1.2 t , U =4.5 t and μ =−2.25 t . Full size image Note that the spatially varying phases in the FF superfluids in both 1D and 2D indicate that there may exist a finite mass supercurrent flow across the system. However, this current is compensated by the backflow of the quasi-particle current arising from the imbalanced spin polarization; therefore, no net mass current is expected [16] . This basic conclusion can also be understood from the fact that net current is determined by J =∂ F ( Q )/∂ Q , where F is the total free energy of the system; therefore, the net current is zero for the ground state. Experimental observations Several different methods may be used to observe both finite-momentum pairing and topological MFs. For instance, the noise correlation of the time-of-flight images [47] may reveal the total momentum of the Cooper pairing of the FF superfluids, which could be quite large in the presence of a suitable in-plane Zeeman field. The momentum-resolved radio-frequency spectroscopy [48] may be used to directly map the quasi-particle band structure of the superfluid, where the asymmetric quasi-particle band dispersion of FF superfluids may be probed [35] , [49] . From Fig. 2 , we see that even for a moderate interaction strength, the bulk quasi-particle energy gap E g may be larger than 0.3 E F , which is much larger than the resolution of the radio-frequency spectroscopy. The large energy gap also ensures that the physics presented here can be observed even at a finite temperature T when T is smaller than the Kosterlitz–Thouless transition temperature, which approaches E F /8 in the strong interaction regime for the gapped system [31] . Moreover, the energy difference per particle between BCS excited state and FF ground state is greatly enhanced by the SO coupling [33] , [35] , [50] ; therefore, the ground state can be reached at proper finite temperature by carefully cooling cold atom gases. Generally, non-FF topological superfluids with zero total momentum pairing can be observed without an in-plane Zeeman field. The optimal parameters for observing topological FF superfluids should be the region with a large energy gap and a large FF momentum. Therefore, relatively large Zeeman fields h x and h z , although not strong enough to destroy the Cooper pairings, are preferred in experiments. Further, the phase transition to the topological superfluid with MFs is accompanied with the bulk quasi-particle excitation gap closing and reopening at k =0, which should also be observable in the momentum-resolved radio-frequency spectroscopy. MFs yield spatially localized zero-energy peak in local density of states [51] , which is separated from other quasi-particle states by a gap at the order of Δ, and can be detected using spatially resolved radio-frequency spectroscopy [52] . Because of the lack of disorder and the precisely controlled experimental parameters in cold atoms, the momentum and spatial resolved radio-frequency spectroscopy measurements should provide conclusive signature for topological FF superfluids with MFs. Our proposed topological FF phase may also be realized using semiconductor/superconductor heterostructures. Recently, topological BCS superconductors and the associated MFs have been proposed in such heterostructures [5] , [6] , [7] , [8] and some preliminary experimental signatures have been observed [11] , [12] , [13] , [14] . To realize a topological FF superconductor, the semiconductor should be in proximity contact with a FF superconductor, which introduces finite-momentum Cooper pairs. The topological parameter region defined in equation (5) still applies except that the order parameter, chemical potential and FF vector are external independent parameters. The flexibility of equation (5) makes it easier for tuning to the topological region with MFs. Because the FF state can sustain in the presence of a large magnetic field, it opens the possibility for the use of many semiconductor nanowires with large SO coupling but small g -factors (for example, GaSb, hole-doped InSb and so on). In summary, we propose that topological FF superfluids or superconductors with finite-momentum pairings can be realized using SO-coupled s -wave superfluids subject to Zeeman fields and they support exotic quasi-particle excitations such as chiral edge modes and MFs. The phase transition to the topological phases depends strongly on all physical quantities, including SO coupling, chemical potential, Zeeman field and its orientations, paring strength, FF vector Q and the effective mass of Cooper pairs explicitly, which are very different from topological BCS superfluids/superconductors that are intensively studied recently. These new features not only provide more knobs for tuning topological phase transitions, but also greatly enrich our understanding of topological quantum matters. The topological FF phases have not been discussed before, and the phases unveiled in this article represent a totally new quantum matter. After the submission of this manuscript, we become aware of relevant work [53] , where topological FF phases in 2D are discussed using slightly different SO coupling and Zeeman field. Momentum space BdG equations The partition function at finite temperature T is , where with H defined in equation (1), and in real space. The FF phase is defined as follows: where Q is the total momentum of the Cooper pairs and Δ is a spatially independent constant. Here, the position-dependent phase of Δ( x ) can be gauged out by the transformation ψ σ → ψ σ e i Q . x /2 . Integrating out the fermion field ψ and ψ † , we obtain , with effective action where β =1/ T , and G −1 =∂ τ + H BdG . The order parameter, chemical potential and FF vector Q are determined self-consistently by solving the following equation set where Ω= S eff / β is the thermodynamical potential. In our model, the deformation of Fermi surface is along the y direction, thus we have Q =(0, Q y ), and only three parameters need be determined self-consistently. In practice, the ground-state phase diagram of the system (that is, Δ, μ , Q y ) is determined by the saddle point of Ω, which can be obtained by minimizing the free energy F ( Q )=Ω+ nμ with respect to these parameters. In our self-consistent numerical calculations, we also compare the free energies for FF superfluids (let Q y as a variable) and normal BCS superfluids (enforce Q y =0), and find that SO coupling generally increases the energy difference between FF ground states and BCS excited states [33] , [35] , [49] , [50] . The energy difference per particle is for a 2D Fermi gas, which ensures that the predicted exotic states may be observable in experiments at finite temperature. We determine different quantum phases using the following criterion. When E g >0, Δ ≠ 0, we have gapped FF phases ( =−1(=+1) for topological, and =+1 (=0) for non-topological state). When there is a nodal line with E g =0 and Δ ≠ 0, we have gapless FF phases. When Δ=0 (then Q =0 is enforced), we get normal gas phases. It is still possible to observe gapless excitations in the gapless FF phase regime; however, we do not distinguish this special condition because gapless excitations are not protected by gaps. In our numerics, the energy and momentum are scaled by Fermi energy E F and its corresponding momentum K F in the case without SO coupling and Zeeman fields. The results in Figs 2 and 3 are determined at and T =0. Real-space BdG equations In the tight-binding model of equation (6), the many-body interaction is decoupled in the mean-field approximation. The particle number and superfluid pairing Δ i = − U c i ↓ c i↑ are determined self-consistently for a fixed chemical potential. Using the Bogoliubov transformation, we obtain the BdG equation where with f ( E )=1/(1+ e E / T ) is the Fermi–Dirac distribution function. In the tight-binding model, the FF phase and the LO phase can be determined naturally, which depend crucially on the parameters of the system as well as the position of the chemical potential [37] . The results in Figs 4 and 5 are obtained at T =0. Topological boundaries in lattice models To determine the topological phase transition conditions, we transform the tight-binding Hamiltonian to the momentum space in equation (2). Here ξ k is replaced by −2 t cos( k x )−2 t cos( k y )− μ for the kinetic energy, and k α by sin( k α ) for the SO coupling, where α = x , y . The topological boundary conditions can still be determined by the Pfaffian of Γ( K )= H BdG ( K )Λ at four non-equivalent points, K 1 =(0,0), K 2 =(0, π ), K 3 =( π , 0), K 4 =( π , π ) when the system is gapped. At these special points, Γ( K ) is a skew matrix. The topological phase is determined by For uniform BCS superfluids, the Pfaffian at K 2 and K 3 are identical, thus only K 1 and K 4 are essential to determine the topological boundaries. However, in our system, all four points affect the topological boundaries, and the exact expression of is too complex to present here. In 1D chain, there are only two non-equivalent points at K 1 =0 and K 2 = π . We find Pf(Γ( K 1 ))=Δ 2 −( h z − μ −2 t cos( Q y /2))( h z + μ +2 t cos( Q y /2))−( h x + α sin( Q y /2)) 2 , and Pf(Γ( K 2 ))=Δ 2 −( h z − μ +2 t cos( Q y /2))( h z + μ −2 t cos( Q y /2))−( h x − α sin( Q y /2)) 2 . The topological index in the gapped regime is determined by How to cite this article: Qu, C. et al. Topological superfluids with finite-momentum pairing and Majorana fermions. Nat. Commun. 4:2710 doi: 10.1038/ncomms3710 (2013).